Realizing a robust practical Majorana chain in a quantum-dot-superconductor linear array Semiconducting nanowires in proximity to superconductors are promising experimental systems for realizing the elusive Majorana fermions, which, because of their non-Abelian anyonic braiding statistics, may ultimately be used as building blocks for topological quantum computers. A serious challenge in the experimental realization of the Majorana fermions is the suppression of topological superconductivity by disorder together with the tunability of carrier density for semiconductors in close proximity to superconductors. Here we show that Majorana fermions that are protected by a disorder robust topological gap can occur at the ends of a chain of gate-tunable quantum dots connected by s -wave superconductors. Such an array of quantum dots provides the simplest realization of Majorana fermions in systems as simple as a few quantum dot array. The proposed system provides a very practical and easily realizable experimental platform for the observation of non-Abelian Majorana modes. Solid-state Majorana fermions (MFs) with non-Abelian statistics are the most promising candidates for realizing systems with a topologically degenerate ground state. Such particles have attracted recent attention both owing to their fundamental interest as a new type of particle with non-Abelian statistics and their potential application in topological quantum computation [1] , [2] , [3] , [4] , [5] , [6] . Over the past few years, it has been realized that topological superconductors provide one of the conceptually simplest platforms for the solid-state realization of MFs. More recently, it was shown that topological superconductors with MFs can occur fairly generically in systems containing the three ingredients of conventional s -wave superconductivity, time-reversal breaking (for example, via a magnetic field), and spin–orbit coupling [7] , [8] . A simple topological superconducting (TS) system supporting MFs, which has attracted serious experimental attention [4] , [5] , consists of a semiconductor nanowire in a magnetic field placed on an ordinary superconductor [9] , [10] . The s -wave proximity effect on an InAs quantum wire, which also has a sizable SO coupling, has already been realized in experiments [11] , and the search for the corresponding TS phase, in the presence of a magnetic field, with localized Majorana modes in semiconductors, is actively being pursued in many laboratories worldwide. The theoretical demonstration [12] that such 1D systems can show non-Abelian statistics has made these systems viable components for quantum information processing. While the proposal for the realization of MFs in semiconductor structures has generated considerable theoretical interest and even inspired significant experimental efforts (refs 13 , 14 , 15 , 16 ; C.M. Marcus, personal communication; J.M. Martinis, personal communication; and G. Gervais, personal communication), a few key challenges relating to non-idealities in realistic systems remain. One such practical challenge is whether it is possible to control the chemical potential of a semiconductor wire, which is absolutely essential to tune the system into the TS phase, because it is in contact with a superconductor [17] . The other key challenge arises from the fact that the TS gap is typically suppressed by strong disorder [18] , [19] , [20] , [21] , [22] , [23] , [24] , [25] . Therefore, the present proposals for realizing MFs would either require clean semiconductor systems or a spin–orbit coupling that is large enough to dominate over the disorder scattering effects [18] , [19] , [20] , [21] , [22] , [23] , [24] , [25] . It is completely unclear at this stage whether these key obstacles of chemical potential tuning and low disorder can be overcome in the currently studied semiconductor nanowire structures, unless substantial materials development occurs first. Our proposal in this paper overcomes both of these problems completely in one stroke by coming up with a new architecture (that is, topology) for creating the Majorana fermion. Additionally, our proposal involves using semiconductor quantum dots coupled to superconducting grains, which is in many ways a simpler system to work with than the earlier two-dimensional (2D) [7] , [8] or one-dimensional (1D) structures [9] , [10] for observing the TS phase. We are fairly confident that the system proposed in the current paper is by far the most ideal experimental platform to search for the solid-state Majorana modes. The simple practical system we propose is composed of a linear quantum-dot(QD)/superconductor (SC) array (shown in Fig. 1a ) to realize the non-Abelian MF modes at the ends of the array. The effects of disorder in the QD/SC array are suppressed in a transparent way, because the topological state can be formed as long as the electron can hop from one QD to a neighbouring QD in the array, which is a much easier condition to satisfy than the near ballistic transport condition necessary through a wire. We emphasize that all that is needed here is for any pair of neighbouring QDs to have finite electronic wavefunction overlap that is, nearest-neighbour hopping through the SC islands—no overall coherence among all the QDs is necessary. Strong disorder can typically renormalize the hopping across QD or SC islands; however, as long as the disorder energy scale is less than the fermi energy, one can choose the length of the QD or SC islands to be shorter than the localization length to enable significant transmission probability. We mention that the number of electrons per dot (they could be as few as a few 10 s), whether the dots are identical or not, whether hopping through the whole linear array is coherent or not, how many dots there are in the system (as few as 5–10 or even fewer depending on the level of noise), the Coulomb charging energy for the QD are all non-issues for the realization of the TS phase (as we have explicitly verified numerically)—the only constraints are that there should be only one electron at the chemical potential in each dot (which can be secured by adjusting the local gates individually on each dot) and there should be enough nearest-neighbour hopping to ensure local proximity effect. Our proposal provides a direct way to see how a zero-energy state, which is fine-tuned to zero becomes topologically robust as more dots are added to the chain. Thus, in this proposal the initial signatures of a zero-energy state can even be seen with as few as a single QD or just three QDs. Our proposal works both for electron and hole QD systems as long as SC proximity effect exists. 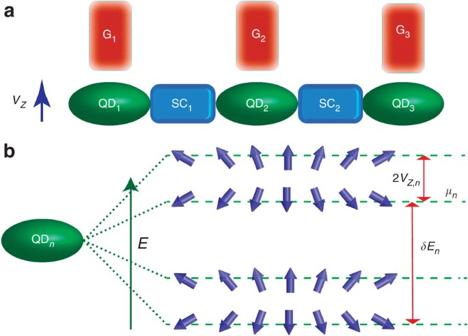Figure 1: Geometry to create disorder robust TS systems with end MFs using a QD–SC array. (a) In the appropriate parameter regime non-Abelian MFs are predicted to occur and be localized at the end QDs of a disordered QD/SC array. Each QD/SC island in the array has a different index to indicate that each QD or SC can have a different local disorder potential, hopping amplitude or proximity-induced superconducting pairing potential. The chemical potentialμnin each QD is controlled by the gateGn. Tunnelling through the superconductor is assumed to be weaker than the magnetic field induced Zeeman splittingVZ,n∼VZof the QD levels. Applying fluxes to the SC islands can compensate relative signs between anomalous and normal tunnelling. (b) Level structure of thenth QD relative to the fermilevel (shown by a dashed line). The level spacingδEnis assumed to be the largest energy scale (∼2–3 meV), the spin splitting 2VZ,nis of the order∼0.3 meV. The gate potentials are tuned to bring the chemical potentialμnto be resonant with the fermilevel in the SC. The spin texture in each level, which is a result of spin–orbit coupling and is determined by the length of the QD relative to the spin–orbit lengthlSO, has a crucial role in allowing spin-singlet proximity-effect between different QDnand QDn+1. This qualitative features of the level structure are independent of local disorder potential. Figure 1: Geometry to create disorder robust TS systems with end MFs using a QD–SC array. ( a ) In the appropriate parameter regime non-Abelian MFs are predicted to occur and be localized at the end QDs of a disordered QD/SC array. Each QD/SC island in the array has a different index to indicate that each QD or SC can have a different local disorder potential, hopping amplitude or proximity-induced superconducting pairing potential. The chemical potential μ n in each QD is controlled by the gate G n . Tunnelling through the superconductor is assumed to be weaker than the magnetic field induced Zeeman splitting V Z , n ∼ V Z of the QD levels. Applying fluxes to the SC islands can compensate relative signs between anomalous and normal tunnelling. ( b ) Level structure of the n th QD relative to the fermilevel (shown by a dashed line). The level spacing δE n is assumed to be the largest energy scale ( ∼ 2–3 meV), the spin splitting 2 V Z , n is of the order ∼ 0.3 meV. The gate potentials are tuned to bring the chemical potential μ n to be resonant with the fermilevel in the SC. The spin texture in each level, which is a result of spin–orbit coupling and is determined by the length of the QD relative to the spin–orbit length l SO , has a crucial role in allowing spin-singlet proximity-effect between different QD n and QD n +1 . This qualitative features of the level structure are independent of local disorder potential. Full size image QD–SC array The confinement potential of the QD separates the electronic energy levels in the dots as shown in Fig. 1b , so that there are two levels (because of time-reversal symmetry induced Kramers-degeneracy). For clean TS systems, it is known that gapped superconductors are topological as long as they have an odd number of occupied bands at the fermilevel [9] , [10] , [26] . To realize a TS QD/SC array, the Kramer-degeneracy of the levels must be broken so that an odd number of occupied levels per QD occurs at the fermi level. The Kramer's degeneracy can be lifted, as shown in Fig. 1b, by breaking time-reversal symmetry by an externally applied magnetic field-induced Zeeman splitting V Z . Disorder in the QD affects the wavefunction and causes fluctuations in the spacing of the levels in the dots, but does not affect the qualitative structure shown in Fig. 1b . In the limit where the QD/SC tunnelling t (which is physically characterized by the inverse tunnelling time from QD to SC) is small compared with the Zeeman splitting between the spin-split levels, the chemical potential can be adjusted by using gate voltages ( Fig. 1a ), so that only a single level in each QD participates in transport through the QD/SC array structure. As only a single spin-polarized level in the QD is resonant with the fermilevel of the SC, double occupancy of the QD is forbidden by Pauli exclusion principle and Coulomb blockade effects are expected to be small. As in the TS phase of other [7] , [8] , [9] , [10] superconductor-semiconductor structures, spin–orbit coupling has a crucial role in determining the superconducting gap in the TS phase. Because the single levels in each QD are spin-polarized almost in the same direction, spin–orbit coupling is necessary to lead to a rotation of the spin-polarization between the left and right end of the QD ( Fig. 1b ) so as to allow a proximity-induced SC coupling between neighbouring QDs. The on-site proximity-induced SC coupling in the same QD is forbidden by the Pauli exclusion principle. Thus, one can expect that the QD–SC chain is equivalent to a 1D lattice model with a single spin-polarized fermionic state per site, together with normal and anomalous hoppings, which may be random. A more detailed derivation of this model, hereafter referred to as the disordered Kitaev chain, is provided in the Methods section. Disordered Kitaev chain In the limit of weak (compared with level spacing in the QD) QD/SC tunnelling together with a chemical potential so that a single non-degenerate spin-split level is present at the fermilevel, the low-energy part of the BdG quasiparticle spectrum in this system, containing the zero-energy Majorana modes in the TS phase, can be described in terms of an effective 1D Kitaev chain [26] lattice-model where is the creation operator in the active level in each QD, μ n the effective chemical potential in each QD, t n and Δ n are the normal and anomalous tunnelling amplitudes between the QDs. The effective proximity-induced superconducting pairing amplitude Δ n depends on the spin-rotation along the QD, shown in Fig. 1b, and the quantitative estimation of Δ n together with a discussion of realistic parameters for InAs QDs is presented in the Supplementary methods . In a disordered QD/SC array, the amplitudes t n , Δ n would vary along the length of the chain, whereas the chemical potential μ n should be gate-tunable to be nearly zero. Thus, the system we are proposing is not really a coherent 1D nanowire, as in the original theoretical proposal of Kitaev [26] or in the recent concrete proposals involving 1D semiconductor nanowires [9] , [10] . Sign-ordered Kitaev chain The effective Kitaev chain description of the QD/SC array allows us to reduce the complexity of an array of disordered QDs and SCs to just three parameters μ n , t n , Δ n for each QD. Furthermore, the complex conjugation symmetry of the full BdG Hamiltonian for the QD–SC system containing pure Rashba spin–orbit coupling can be shown to result in real effective parameters, t n and Δ n . In the perfectly periodic case where the amplitudes t n and Δ n and the local potential μ n are independent of n , the topological condition, which allows one to realize a TS phase with MFs, is given by | μ n |<| t n | (ref. 26 ). In a disordered QD/SC array, the magnitudes of t n may be controlled, in principle to a certain degree by controlling the QD/SC tunnelling. However, the magnitude of Δ n or the signs of t n , Δ n are more difficult to control given the disorder in the SC islands and the short fermi wave vectors of electrons in the SC islands. Whereas the phases (or signs) of the hopping amplitude t n can be chosen using a gauge transformation such that t n >0, the pairing amplitude Δ n can have random phases (which are restricted to 0, π for purely Rashba SO coupling), which cannot be removed by a gauge transformation and thus have physical consequences. Even for an otherwise clean Kitaev chain (that is, with μ n , t n independent of n ) in the TS phase, a disorder induced sign-flip of Δ m over a block of sites, creates π -junction domain-walls with pairs of localized zero-energy MF modes [26] . These disorder-induced sign flips of Δ m can be expected to suppress the bulk TS phase gap to zero, unless explicitly avoided. Thus, a strongly disordered Kitaev chain is expected to have a large number of low-energy states, similar to a disordered topological superconductor, hindering the observation of non-Abelian statistics and consequently topological quantum computation. These low-energy states can be eliminated by shifting the phase of the superconducting order parameters on a subset of the SC islands by approximately π (or some other value for non-Rashba spin–orbit coupling), so that the Δ n are real and sgn( t n Δ n )=sgn( t n +1 Δ n +1 ). Because the TS phase of the Kitaev chain is gapped, the TS phase is expected to be robust to small deviations in the phase-shifts. In what follows, we will restrict our discussion to such Kitaev-chains with appropriately tuned superconducting phases, henceforth referred to as sign-ordered. MFs in sign-ordered Kitaev chains In the Supplementary methods, we have shown that a sign-ordered but otherwise disordered Kitaev-chain can be in a TS phase containing end MFs for a broad range of parameters. In particular, we find that such a QD chain containing an odd number of sites always supports a pair of localized zero modes if the chemical potential, μ n , at each site can be tuned to μ n =0 and the hopping amplitudes are sign-ordered. Even a single QD coupled to a superconductor has a zero-mode when its chemical potential is tuned to the fermilevel, though this degeneracy is not associated with spatially separated MF modes. Physically, this is because hopping and superconductivity cannot have an effect on a single spin-polarized site, so one expects that tuning the chemical potential to be resonant with the superconductor produces a zero-energy state (relative to the superconductor). A degeneracy associated with spatially separated MF-end modes is obtained for a chain with three QDs with μ n =0 and t 1 =Δ 1 and t 2 =Δ 2 . The degeneracy associated with spatially separated localized MF modes in the chains with μ n =0 is topologically protected against fluctuations in the chemical potential μ n away from zero because of fermion parity [7] , [8] , [26] . In fact, in the Supplementary methods , using a transfer matrix formalism similar to ref. 27 , we show that the general (that is, with μ n ≠0) sign-ordered Kitaev chain has a chiral symmetry and therefore supports a TS phase with robust end MFs whenever a corresponding non-Hermitean Hamiltonian is in the delocalized phase [28] , [29] . The MF modes are thus found to be exponentially localized and protected whenever where the expectation value is taken with respect to the random distribution for the magnitudes of | t n |, |Δ n | and is the localization length of an effective Hermitean Hamiltonian with on-site potential μ n and hopping . Here | ζ | −1 turns out to be the localization length of the MF. The parameter regime ζ <0 supporting end MFs, which defines the topological phase of the MF Hamiltonian, corresponds to the delocalized phase of an effective non-Hermitean Hamiltonian, whereas the complementary parameter regime defining the non-TS phase corresponds to the localized phase [28] , [29] . Furthermore, in the Supplementary methods, we provide a detailed discussion of why the sign-ordered Kitaev chain with the Hamiltonian in equation (1) remains gapped for otherwise arbitrary disorder under this condition. Whereas the analytic results provide some understanding of how zero-energy MF arise in the sign-ordered Kitaev chain, it is more insightful to consider the spectra of typical realization of finite sign-ordered Kitaev chains. We consider, in Fig. 2, the spectrum of a five-site (we have used several different number of sites in our numerical work getting the same qualitative answer) Kitaev chain with open boundary conditions. Choosing realistic random values for μ n (with mean μ n =0), t n and Δ n , which vary over a significantly larger range then their minimum values, we find a robust TS phase with end MFs, which appear as zero-energy eigenstates. The end MFs are not strictly localized at the ends of the chain, but are split by an exponentially small amount due to overlap of the decaying MF wavefunctions across the chain. The exponential dependence on the chain length of the energy splitting, seen in Fig. 3, shows clearly the exponential localization of the MFs and also demonstrates that the protection of the topological degeneracy of the MFs increases exponentially with the length of the chain. An interesting feature from setting the gate potential to be near μ n =0 is that the MF splitting decreases exponentially starting with a value proportional to the fluctuations of μ n . Therefore, nearly zero-energy subgap modes can be obtained in the QD/SC array case even for short chains, if the gate voltages can be tuned sufficiently precisely. 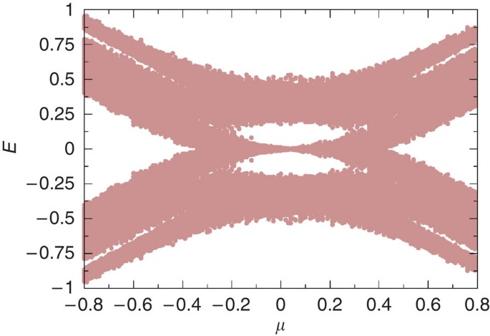Figure 2: Spectrum of a disordered 1D Kitaev chain of lengthN=5 sites. The hopping amplitudestand pairing amplitudes Δ are distributed randomly and uniformly in the interval [0.5,1.5] K. The chemical potentialμis taken to have a mean value, which varies from −4.0 to 4.0 K, and a site to site fluctuation of 250 mK. The spectrum shows a near-zero-mode separated by a gap∼1 K in a range of on-site QD chemical potential. Thus, the TS state shows a robust gap in this regime despite the large fluctuations in the hopping, pairing potential and chemical potential. The level broadening of the zero-mode is a result of the finite length of the chain together with the disorder fluctuations. Figure 2: Spectrum of a disordered 1D Kitaev chain of length N =5 sites. The hopping amplitudes t and pairing amplitudes Δ are distributed randomly and uniformly in the interval [0.5,1.5] K. The chemical potential μ is taken to have a mean value, which varies from −4.0 to 4.0 K, and a site to site fluctuation of 250 mK. The spectrum shows a near-zero-mode separated by a gap ∼ 1 K in a range of on-site QD chemical potential. Thus, the TS state shows a robust gap in this regime despite the large fluctuations in the hopping, pairing potential and chemical potential. The level broadening of the zero-mode is a result of the finite length of the chain together with the disorder fluctuations. 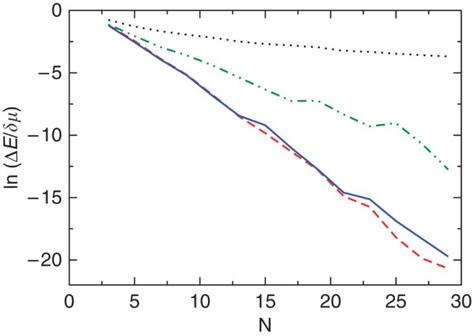Figure 3: Finite size splitting ΔEof Majorana modes as a function of chain length for differentδμ. Dashed red line:δμ=250 mK; solid blue lineδμ=500 mK; dotted-dashed green lineδμ=1.5 K; black dotted lineδμ=2.5 K. Finite chain length leads to overlap of end MFs, which splits them away from zero energy in any finite system. The MF splitting ΔEin the disordered 1D Kitaev chain (with the same parameters as inFig. 2) is proportional to and always less than the fluctuation of chemical potentialδμand is found to go to zero exponentially in odd-number-chain lengthN. The localization length of the MF becomes shorter for less disordered chains. Full size image Figure 3: Finite size splitting Δ E of Majorana modes as a function of chain length for different δμ . Dashed red line: δμ =250 mK; solid blue line δμ =500 mK; dotted-dashed green line δμ =1.5 K; black dotted line δμ =2.5 K. Finite chain length leads to overlap of end MFs, which splits them away from zero energy in any finite system. The MF splitting Δ E in the disordered 1D Kitaev chain (with the same parameters as in Fig. 2 ) is proportional to and always less than the fluctuation of chemical potential δμ and is found to go to zero exponentially in odd-number-chain length N . The localization length of the MF becomes shorter for less disordered chains. Full size image In conclusion, the two major problems of the semiconductor–superconductor structures, proposed [7] , [8] , [9] , [10] in the context of creating non-Abelian solid-state Majorana modes, are disorder and gating. Both problems are solved by using the relatively simple QD/SC linear array structure shown in Fig. 1 . Although the operation of this linear array in the clean limit is qualitatively similar to the semiconductor nanowire proposals [7] , [8] , [9] , [10] , the behaviour in the presence of disorder is qualitatively different. In particular, for the reasonable model of disorder chosen, the QD/SC array continues to have a robust quasiparticle gap, whereas the semiconductor nanowires are expected to almost completely lose the quasiparticle gap [23] , [24] . Part of the origin of this robustness is the fact that the use of QDs allows one to control the chemical potential locally by gates (thus eliminating the gating problem), which is fundamentally impossible with impurities in nanowires. However, this neccessitates the use of SC grains, which can potentially introduce random π junctions in the chain that can produce subgap states. These effects of strong disorder are avoided by adding an array of gates and removing accidental π junctions by phase shifting the superconductors. Furthermore, MFs have been shown to be robust to weak Coulomb interaction effects [30] , [31] , [32] . Finally, structures similar to the QD/SC array being proposed in this work are already in use in various conventional quantum computing architectures such as quantum dot spin qubits and superconducting Cooper-pair box qubits, thus making this a relatively practical (as well as extremely robust) proposal for creating non-Abelian modes in the laboratory. In hindsight, the origin of zero-modes in the QD array is the conceptually simplest among all the proposals for MFs [7] , [8] , [9] , [10] and can be traced to the fact that the energy level of a single QD, which is the single-site limit of the proposed QD/SC array, can always be tuned by a gate voltage to have a zero mode and is always robust to disorder. It is interesting to speculate why this simple idea (that is, robust QD/SC MF) followed rather than preceding the more complex and less robust 2D [7] , [8] and 1D [9] , [10] MF proposals. One possible reason for the late arrival of the rather obvious idea of the simple QD/SC platform as the non-Abelian MF host may be purely historical with the subject following the early lead of the proposed 2D fractional quantum Hall qubit [33] and 1D Majorana Kitaev chain [26] . The surprising result obtained in this paper is that these zero modes evolve into the the topological MF modes, whose degeneracy becomes exponentially robust with increasing number of sites in the chain. The fact that only a few semiconductor QDs (perhaps as few as three) are necessary (and either electron or hole dots could be used) for the realization of a robust non-Abelian Majorana mode makes our proposal highly attractive from the experimental perspective. Deriving the effective Kitaev Hamiltonian for the QD–SC array In this section, we derive equation (1), which is the effective Kitaev chain model [26] starting from the BdG Hamiltonian for a coupled QD–SC system. This is done in the two steps discussed in the subsections below. In the first subsection, we determine the structure of the energy levels and the wavefunctions in the QDs. We show that, in a certain parameter regime, one needs to only consider a single fermionic level for each QD, and therefore, the BCS Hamiltonian can be thought of as a tight-binding model similar to the Kitaev chain. We also discuss the constraints on the size of the QDs, spin–orbit coupling, and so on, and show that these parameters are reasonable for InAs QDs. In the next section, we derive the tunnelling t n and pairing amplitude Δ n terms between these levels by considering matrix elements between the wavefunctions derived in the first subsection. Spin–orbit coupled QDs We start by discussing the interplay of confinement, Zeeman splitting, spin–orbit coupling, and disorder in determining the wavefunction of the active level in the QD in the vicinity of the fermilevel. Such an understanding is obtained by considering a Rashba spin–orbit coupled 1D system with a Hamiltonian where m * is the semiconductor effective mass, V Z is the magnetic-field induced Zeeman potential, V ( x ) represents the combination of the confinement potential and local disorder potential and α is the strength of the Rashba spin–orbit coupling. We have approximated the QD to be 1D, because the confiment energy of the QDs along the transverse direction can be as large as ∼ 40 meV (refs 34 , 35 ). The Rashba spin–orbit coupling leads to a variation of the local spin-density along the axis x of the QD, which can be described by transforming each eigenstate according to a spin-dependent gauge transformation where is the effective spin–orbit length, which is the length travelled by an electron before it precesses by π under the influence of the spin–orbit magnetic field. Substituting this into the Schrodinger equation, we find that the spin–orbit term can be completely eliminated in this new basis, so that the new Schrodinger equation is written as Ignoring the relatively small Zeeman splitting ( V Z ∼ 0.5 meV), the energy splitting for levels in the QD , where is the mean fermi veloctiy at an energy E relative to the bottom of the band and 2 a is the length of the QD. As the energy E must be less than the inter sub-band separation ∼ 40 meV, we choose E ∼ 5 meV, so that δE ∼ 3 meV for a QD of length 2 a ∼ 120 nm, using the example of InAs electron systems [11] , where the SC proximity effect has been realized. In the absence of a Zeeman splitting (that is, V Z =0), the energy levels in the QD, which are separated by around δE ∼ 3 meV on average, are two-fold degenerate owing to time-reversal symmetry. Disorder potentials can lead to statistical variations in the spacings of the QD levels. However, by tuning the gate voltage of the QD, it should be possible to tune to a pair of levels that are separated from other levels by the average separation of δE ∼ 3 meV. While the disorder potential in the QD is allowed to be large, we will assume that the length of the QD, 2 a , is not significantly longer than the mean-free path so that the spatial part of the wavefunction ψ 0 ( x ) of the pair of levels in the QD extends over the entire length of the QD. This assumption is valid in realistic systems. As V Z ∼ 0.5 meV ≪ δE =3 meV, the effect of V Z can be treated as a perturbation splitting the twofold degeneracy of the pair of states at the fermi level. For a < l SO , the Zeeman field perturbation proportional to V Z in equation (5) in the degenerate space is given by an effective magnetic field for the pair of states at the fermi level. The Zeeman field splits the degenerate pair of levels into non-degenerate levels separated by , which we take to be larger than meV for a < l SO . Moreover, the wavefunction of the lower spin-split state is where . Substituting back the wavefunction into equation (4), we obtain the approximate expression for the wavefunction of the active state in the QD where σ =±1 are eigenstates of σ z . The realization of MFs in the QD system requires the introduction of the superconducting proximity effect from neighbouring s -wave SC islands. Superconducting proximity effect and tunnelling Let us now consider how the proximity effect can by induced from the SC islands in the QD/SC chain. As the states in the SC are gapped, we can integrate out the states in the SC and replace the SC by an effective Hamiltonian [36] , which is schematically written as where E ≪ Δ (Δ being the superconducting gap in the SC island) is the BdG quasiparticle energies, we are solving for, G SC is the effective superconductor Green function and t is the tunnelling between the QDs and the SCs. The Green-function of the SC (for uniform Δ), even in the presence of disorder, is written as where φ n ( x ) are the spatial parts of the electronic eigenstates with energy ɛ n relative to the fermilevel in the normal state of the SC island and we have used the choice ( u ↑ ( x ), u ↓ ( x ), v ↓ ( x ), − v ↑ ( x )) T for the Nambu spinor so that the BdG Hamiltonian for the s -wave superconductor is spin-independent. Here u σ ( x ) and v σ ( x ) are the electron and hole part of the BdG quasiparticle wavefunctions. The qualitative form for G SC is valid even for strongly disordered s -wave superconductors and the only role of strong disorder in the SC islands is to reduce the coherence length of the superconductor, which limits the width of the SC because the SC island is required to be shorter than the coherence length so that the matrix elements of ∑ SC ∝ G SC ( xx ′) is non-vanishing between neighbouring QDs. In particular, for states at energies much smaller than the quasiparticle gap Δ in the superconductors, one can assume E ∼ 0, so that G SC ( E ∼ 0) is particle-hole symmetric, Hermitean and spin-independent. The effective self-energy induced by the superconductor in coordinate (that is, x , x ′) space can be written as a spin-independent sum of a normal and anomalous part as where are the normal and anomalous components of the self-energy. Here the matrices τ x , y , z are Pauli matrices in the Nambu space containing the particle-hole degrees of freedom. To calculate the effective BdG Hamiltonian in the subspace of the low-energy (that is, near the fermilevel at E ∼ 0) active levels in each QD, we note that the low-energy basis of the n th QD consists of an electron-like wavefunction described by an x -dependent 4-component spinor wavefunction Ψ e , n ( x )=( ψ n ( x ), 0) T and a hole wavefunction (since ψ n ( x ) is real), where ψ n ( x ) is the position dependent 2-component spinor wavefunction of the active level in the QD given by equation (6). The iσ y matrix flips the spin of the electron spinor relative to the holes.Taking the relevant matrix elements of the tunnelling operator t of the n th SC island between the right end of the n th QD and the left end of the ( n +1)th QD we find that the effective normal tunneling between QD n and QD n +1 is given by where we have used the QD wavefunctions from equation 6 and is the spatial part of the matrix element of the QD wave-function with the superconducting self-energy . Similarly, the anomalous hopping or cross-Andreev reflection amplitude induced between the dots is given by where is the spatial part of the matrix element of the QD wavefunction with the superconducting self-energy . In the limit of weak barrier transparency, when the tunnelling matrix elements are tuned to be of order ≲ Δ, we expect the matrix elements to be of order of the tunnelling matrix elements [36] , which can be made of order Δ. That combining the above equation with equation (6), leads to the fact that, in the limit of vanishing Rashba spin–orbit coupling α , l SO diverges, leading to a vanishing η n and therefore Δ n . Thus, the anomalous hopping amplitude Δ n is proportional to the spin–orbit coupling. An analogous calculation leads to the conclusion that the on-site contribution (that is, from QD n to QD n ) of the anomalous self-energy vanishes, whereas the on-site contribution of the normal self-energy just renormalizes μ n by an amount that can be off-set by changing the gate voltage on gate n . How to cite this article: Sau, J. D. et al . Realizing a robust practical Majorana chain in a quantum-dot-superconductor linear array. Nat. Commun. 3:964 doi: 10.1038/ncomms1966 (2012).